Raman fingerprint of two terahertz spin wave branches in a two-dimensional honeycomb Ising ferromagnet Two-dimensional (2D) magnetism has been long sought-after and only very recently realized in atomic crystals of magnetic van der Waals materials. So far, a comprehensive understanding of the magnetic excitations in such 2D magnets remains missing. Here we report polarized micro-Raman spectroscopy studies on a 2D honeycomb ferromagnet CrI 3 . We show the definitive evidence of two sets of zero-momentum spin waves at frequencies of 2.28 terahertz (THz) and 3.75 THz, respectively, that are three orders of magnitude higher than those of conventional ferromagnets. By tracking the thickness dependence of both spin waves, we reveal that both are surface spin waves with lifetimes an order of magnitude longer than their temporal periods. Our results of two branches of high-frequency, long-lived surface spin waves in 2D CrI 3 demonstrate intriguing spin dynamics and intricate interplay with fluctuations in the 2D limit, thus opening up opportunities for ultrafast spintronics incorporating 2D magnets. The recent discovery of two-dimensional (2D) ferromagnetism [1] , [2] proves that magnetic anisotropy can overcome thermal fluctuations and stabilize long-range magnetic orders in the 2D limit at finite temperatures. This has immediately triggered tremendous interest [3] , [4] , [5] , [6] , [7] , [8] , [9] , [10] , [11] , [12] in potential 2D magnet-based applications, ranging from ultrathin magnetic sensors to high-efficiency spin filter devices. Naturally, a complete description of the 2D magnetic phase is now needed, which requires not only the identification of the ordered ground state, but equally important, the understanding of the excitations, i.e., spin waves, or equivalently, magnons [13] , [14] . To date, there have been no direct comprehensive experimental studies on the full characteristics of spin waves in these 2D Ising ferromagnets, aside from the quasiparticle excitation spectra from the inelastic tunneling measurements in ref. [11] . A spin wave describes the spin dynamics of magnetic ordering when excited, and its frequency determines the ultimate switching speed of state-of-the-art ultrafast spintronic devices [15] , [16] , [17] , [18] . Generally speaking, the well-established spintronic devices based on Heisenberg ferromagnets have speeds in the gigahertz (GHz) regime due to the weak magnetic anisotropy [19] , [20] , while the speeds of the recently proposed antiferromagnet-based spintronic devices fall into the terahertz (THz) range owing to the exchange interaction between the two sublattices of the antiferromagnets [21] , [22] , [23] . Remarkably, the newly discovered 2D Ising honeycomb ferromagnet CrI 3 possesses both merits for realizing high-frequency spin waves: the strong magnetic anisotropy from the Ising-type spin interactions [24] and the large exchange coupling between the two Cr 3+ sublattices within the honeycomb framework [25] . In this work, we study the spin wave excitations in the 2D Ising honeycomb ferromagnet CrI 3 using polarized micro-Raman spectroscopy. Based on Raman symmetry analysis, we uniquely distinguish two spin wave modes at 2.28 and 3.75 THz from the rest of the optical phonon modes. The doubling of the spin wave mode number is a direct consequence of the underlying non-Bravais honeycomb lattice, while the exceptionally high THz frequency for a ferromagnet reflects the strong magnetic anisotropy and exchange interactions in good agreement with theoretical expectations. From the temperature and thickness dependence of the spin wave characteristics, we show that short-range magnetic correlations are set in prior to the formation of a long-range static magnetic order for every thickness, and that stronger fluctuation effects appear in thinner flakes. Remarkably, we found that the integrated intensities (I. I.) of the two spin wave modes exhibit nearly no thickness dependence, in stark contrast to the fact that the I. I. for all optical phonons scale linearly with their sample thickness, as expected for all bulk modes in quasi-2D-layered materials. This observation on the two spin waves, however, shows striking analogy to the surface modes whose I. I. is independent of the thickness. Moreover, we show that, from more than ten-layer to monolayer CrI 3 , the spin wave frequencies (2.28 and 3.75 THz) and the onset temperatures (45 K) remain nearly constant, while their lifetimes decrease significantly from 50 and 100 ps to 15 ps, but remain an order of magnitude longer than their corresponding spin wave temporal periods. Spin wave dispersion calculations in 2D CrI 3 We first performed the spin wave dispersion relation calculations for the monolayer ferromagnet CrI 3 , in which the Cr 3+ cations form a honeycomb structure with the edge-sharing octahedral coordination formed by six I − anions and the magnetic moment of the two Cr 3+ cations (S = 3/2) per unit cell aligns in the same out-of-plane direction (Fig. 1a ). The minimum model to describe this ferromagnetism in the monolayer CrI 3 is the Ising spin Hamiltonian, \(H = - \frac{1}{2}\mathop {\sum }\limits_{\langle i,j \rangle} \left( {J_{{\mathrm{XY}}}\left( {S_i^{\mathrm{X}}S_j^{\mathrm{X}} + S_i^{\mathrm{Y}}S_j^{\mathrm{Y}}} \right) + J_{\mathrm{Z}}S_i^{\mathrm{Z}}S_j^{\mathrm{Z}}} \right)\) , where \(S_{i(j)}^{{\mathrm{X}}({\mathrm{Y}},{\mathrm{Z}})}\) is the spin operator along the X (Y, Z) direction at the Cr 3+ site i ( j ); J Z and J XY are the exchange coupling constants for the out-of-plane and the in-plane spin components, respectively, and satisfy J Z > J XY > 0 for Ising ferromagnetism; and 〈 i , j 〉 denotes the approximation of the nearest-neighbor exchange coupling. 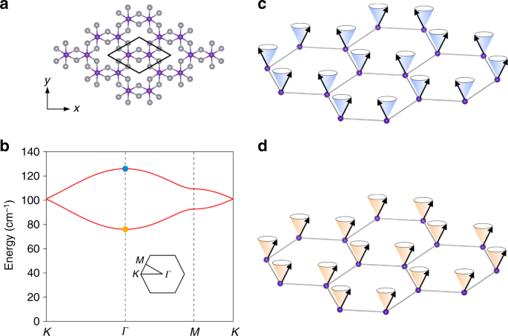Fig. 1 Magnetic excitations in the 2D Ising ferromagnet CrI3.aTop view of the atomic structure of monolayer CrI3, with Cr3+in purple and I–in gray. Cr3+ions form a honeycomb lattice with two Cr3+ions per unit cell (black enclosure).bCalculated magnon dispersion relation in monolayer CrI3. The inset shows the Brillouin zone. Magnon modes at the zone center (Γpoint, zero-momentum) are highlighted by yellow and blue solid circles.c,dSchematic of the zone center magnon modes. The cones represent the precession trajectories of the spins (black arrows). The precession of spins on two Cr3+sublattices are out-of-phase (c) and in-phase (d), which corresponds to the high- and low-energy modes, respectively, inb Figure 1b shows the calculated spin wave dispersion relation along the high-symmetry directions ( Κ–Γ–Μ–Κ ) of the first Brillouin zone (Fig. 1b, inset). Because there are two magnetic Cr 3+ cations per primitive cell, there are two spin wave branches whose eigenstates contain in-phase (lower branch) and out-of-phase (upper branch) spin precessions between the two sublattices [26] . Of particular interest to Raman scattering, as well as the tunneling geometry of the magnetic filter devices, are the spin wave states at the Brillouin zone center ( Γ point, zero-momentum) describing the uniform precession of the spins about the easy axis. The energy barrier from the ground state to the lower branch is proportional to the magnetic anisotropy, \(\Delta _{\mathrm{L}} = \frac{9}{4}\left( {J_{\mathrm{Z}} - J_{{\mathrm{XY}}}} \right)\) , which is the energy cost for the spins to uniformly tilt off the easy axis in this excited state (Fig. 1d ). The energy barrier for the upper branch results from a combined effect of both the magnetic anisotropy and the in-plane exchange coupling, \(\Delta _{\mathrm{U}} = \frac{9}{4}\left( {J_{\mathrm{Z}} + J_{{\mathrm{XY}}}} \right)\) , corresponding to the energy needed for tilting the spins at the two Cr 3+ sublattices in the opposite directions upon this excitation (Fig. 1c ). Fig. 1 Magnetic excitations in the 2D Ising ferromagnet CrI 3 . a Top view of the atomic structure of monolayer CrI 3 , with Cr 3+ in purple and I – in gray. Cr 3+ ions form a honeycomb lattice with two Cr 3+ ions per unit cell (black enclosure). b Calculated magnon dispersion relation in monolayer CrI 3 . The inset shows the Brillouin zone. Magnon modes at the zone center ( Γ point, zero-momentum) are highlighted by yellow and blue solid circles. c , d Schematic of the zone center magnon modes. The cones represent the precession trajectories of the spins (black arrows). The precession of spins on two Cr 3+ sublattices are out-of-phase ( c ) and in-phase ( d ), which corresponds to the high- and low-energy modes, respectively, in b Full size image Raman signature of two sets of zero-momentum spin waves To study both zero-momentum spin waves in 2D CrI 3 crystals, we fabricated CrI 3 thin flakes fully encapsulated by hexagonal boron nitride (hBN) (see sample fabrication details in Methods and thickness characterization in Supplementary Note 1 ) and performed micro-Raman spectroscopy measurements on them as a function of layer number and temperature, as frequency-resolved magnetic Raman scattering cross section is directly proportional to the time-domain magnetic correlation function [27] . In contrast to phonon Raman scattering which preserves time-reversal symmetry (TRS) and thus has symmetric Raman tensors [28] , the leading-order one-magnon Raman scattering involves spin flipping (ΔS = ±1) that breaks TRS, and consequently corresponds to antisymmetric Raman tensors [29] , [30] . Based on the difference in the Raman tensors, we can therefore readily distinguish magnon Raman modes from phonon modes via polarization selection rules. In our Raman measurements with the backscattering geometry, the polarizations of the incident and the scattered light were kept to be either parallel or perpendicular to each other, and could be rotated together with respect to the in-plane crystal axis by any arbitrary angle ϕ . The incident photon energy of 1.96 eV was chosen to be on resonance with the charge transfer and the Cr 3+ 4 A 2 to 4 T 1 transitions of CrI 3 in order to increase the Raman sensitivity of magnon scattering [4] (see Supplementary Note 2 for a comparison with the nonresonant Raman spectra). 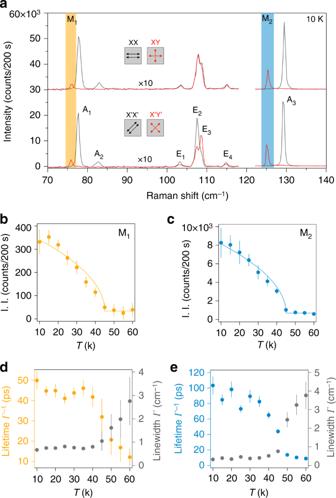Fig. 2 Detection of the zero-momentum magnons in thick CrI3.aRaman spectra of a thick CrI3flake (13 layers) at low temperature (10 K) in the parallel and cross-channels atϕ= 0o(XX and XY) and atϕ= 45o(X’X’ and X’Y’). Magnon modes, M1and M2, appearing only in the cross-channels (XY and X’Y’), are highlighted in yellow and blue. Phonon modes are labeled as A1, A2, E1–E4, and A3. The spectral intensities in the 70–120 cm–1range are multiplied by a factor of 10. The spectra in the XX and XY channels are vertically offset for clarity. The spectra are acquired using a 633-nm excitation laser.b,cTemperature dependence of I. I. of the M1and M2magnon modes, respectively. Solid curves are fits to\(I_0 + I\sqrt {T_{\mathrm{C}} - T}\).d,eTemperature dependence of the lifetime (Γ−1, left axis) and the linewidth (Γ, right axis) of the M1and M2magnon modes, respectively. Error bars inb–erepresent the two standard errors of fitting parameters in the Lorentzian fits to individual temperature-dependent Raman spectra Figure 2a shows low-temperature (10 K) Raman spectra taken on a 13-layer (13 L) CrI 3 flake in both parallel and cross-polarization selection channels at ϕ = 0 o and ϕ = 45 o , denoted as XX, XY, X’X’, and X’Y’, respectively. In total, there are nine Raman-active modes observed, which can be categorized into three groups based on their selection rules. First and most remarkably, the M 1 and M 2 modes are only present in the cross-channels (XY and X’Y’) and are absent in the parallel channels (XX and X’X’) within our detection resolution. This leads to the unique identification of purely antisymmetric Raman tensors for these two modes, evidence of them arising from the two zero-momentum magnons depicted in Fig. 1c and 1d . Of equal interest are their high frequencies at 76 cm –1 (2.28 THz, or 9.4 meV) and 125 cm –1 (3.75 THz, or 15.5 meV), respectively, which are three orders of magnitude higher than those of the conventional ferromagnets used in most spintronic devices today (in the GHz range) [19] , [20] . Even though our measured magnon frequencies are in a similar energy scale as those reported in Ref. 11 (3 and 7 meV, and possibly 17 meV), their quantitative difference is significant and invites further investigations on the spin dynamics in 2D CrI 3 . Furthermore, by substituting Δ L and Δ U with the two magnon frequencies above, the exchange coupling constants for the in-plane ( J XY ) and the out-of-plane ( J Z ) spins are determined to be 11 cm –1 and 44 cm –1 , respectively, in good agreement with that obtained from generalized calculations of magnetic coupling constants for bulk CrI 3 [31] . Second, the A 1 , A 2 , and A 3 modes show up only in the parallel channels (XX and X’X’) without any ϕ dependence, and therefore these are the A g phonon modes under the rhombohedral crystal point group C 3i (space group \(R\overline 3\) ) [32] . Third, the E 1 , E 2 , E 3 , and E 4 modes are the E g phonon modes of C 3i , because of their appearance in both parallel and cross-channels, as well as the rotational anisotropy of their intensities (see detailed analysis for all Raman modes in Supplementary Note 3 ). Fig. 2 Detection of the zero-momentum magnons in thick CrI 3 . a Raman spectra of a thick CrI 3 flake (13 layers) at low temperature (10 K) in the parallel and cross-channels at ϕ = 0 o (XX and XY) and at ϕ = 45 o (X’X’ and X’Y’). Magnon modes, M 1 and M 2 , appearing only in the cross-channels (XY and X’Y’), are highlighted in yellow and blue. Phonon modes are labeled as A 1 , A 2 , E 1 –E 4 , and A 3 . The spectral intensities in the 70–120 cm –1 range are multiplied by a factor of 10. The spectra in the XX and XY channels are vertically offset for clarity. The spectra are acquired using a 633-nm excitation laser. b , c Temperature dependence of I. I. of the M 1 and M 2 magnon modes, respectively. Solid curves are fits to \(I_0 + I\sqrt {T_{\mathrm{C}} - T}\) . d , e Temperature dependence of the lifetime ( Γ −1 , left axis) and the linewidth ( Γ , right axis) of the M 1 and M 2 magnon modes, respectively. Error bars in b – e represent the two standard errors of fitting parameters in the Lorentzian fits to individual temperature-dependent Raman spectra Full size image Temperature dependence of spin waves Having identified the two single-magnon modes in the Raman spectra at low temperature, we proceed to evaluate their temperature dependence. To see the results quantitatively, we fit the magnon modes with a Lorentzian function of the form \(\frac{{A(\varGamma /2)^2}}{{(\omega - \omega _{\mathrm{o}})^2 + (\varGamma /2)^2}}\) , where ω o , Γ , and A are the central frequency, linewidth, and peak intensity of the magnon mode, respectively. Figure 2b, c show the temperature dependence of the I. I., \(\frac{{\mathrm{\pi }}}{2}A\varGamma\) , of the two magnon modes. Clearly, both traces exhibit a clear upturn below a critical temperature T C = 45 K (the same value for bulk CrI 3 ), that is, however, lower than the bulk Curie temperature of 60 K determined by the magnetic susceptibility measurements under a magnetic field of 0.1 T (see the magnetic susceptibility data and Raman data on bulk CrI 3 in Supplementary Note 4 ). The temperature dependence of the magnon lifetimes (inverse of the linewidths, Γ −1 , Fig. 2d, e ), on the other hand, shows that a short lifetime of < 10 ps sets in at 60 K and saturates at about 50 ps (100 ps) around 45 K for the M 1 (M 2 ) magnon. This, together with the divergent behavior of the linewidth temperature dependence (see Fig. 2d, e ), indicates that strong magnetic fluctuations are present before the static magnetic order is established at 45 K. It is therefore likely that 60 K marks the onset of the field-stabilized magnetic correlations, while 45 K denotes the intrinsic transition to the spontaneous ferromagnetism, reconciling the difference between the critical temperatures measured by the two different experimental techniques. This is also consistent with the temperature-dependent magneto-optical Kerr effect [2] and tunneling [7] , [12] measurements of thin samples at zero fields, and explains the difference between the tunneling resistance with [11] and without [7] , [12] a magnetic field appearing above T C . Thickness dependence of spin waves To investigate how thermal fluctuations impact the intrinsic 2D ferromagnetism and its excitations, we performed a systematic Raman study of the M 1 and M 2 magnon modes measured on atomically thin CrI 3 crystals ranging from 13 L to monolayer (1 L). It is clear from the data taken at 10 K in Fig. 3a that both main magnon modes (M 1 and M 2 ) and their satellite modes (highlighted with gray triangles in Fig. 3a ) have a notable layer number dependence. First, the satellite magnon modes arise from the finite thickness effect in thin layers, in which broken translational symmetry perpendicular to the basal plane makes single-magnon modes with finite out-of-plane momenta accessible in Raman scattering [33] , [34] (see the same effect for phonons in Supplementary Note 5 ). The small energy separation between the main mode and the nearest satellite, on the order of 3 cm –1 , indicates the weak interlayer magnetic coupling strength [26] , consistent with the small training magnetic field of less than 1 T reported in literature [2] , [8] , [11] . Moreover, as the layer number decreases, there are fewer but stronger observable satellite magnon modes in the Raman spectra. Second, the two main magnon modes, M 1 and M 2 , persist down to the monolayer with symmetric lineshapes, while their peak intensities drop and their linewidths broaden with decreasing layer numbers. Fig. 3 Layer number dependence of the zero-momentum magnon characteristics. a Raman spectra of the M 1 (intensity multiplied by 20) and M 2 magnons for 1–5 L, 9 L, and 13 L samples. Light yellow and blue shaded areas are the Lorentzian fits for the M 1 and M 2 magnon modes, respectively. The gray triangles highlight the satellite magnon peaks. b Frequency ( ω 0 , left axis) and lifetime ( Γ –1 , right axis) of the M 1 magnon as a function of layer number. c I. I. of the M 1 magnon as a function of layer number with I. I. of the A 1 phonon shown in gray for comparison. d , e Plots for M 2 that are similar to b , c , with I. I. of the A 3 phonon plotted in gray in e for comparison. Error bars in b – e represent the two SEs of fitting parameters in the Lorentzian fits to individual Raman spectra at different thicknesses Full size image To understand the layer number dependence of the M 1 and M 2 magnons in greater detail, we extracted the magnon mode frequencies ( ω o ), lifetimes ( Γ −1 ), and I. I. ( \(\frac{{\mathrm{\pi }}}{2}A\varGamma\) ), from fitting their Raman spectra with the Lorentz function ( \(\frac{{A(\varGamma /2)^2}}{{(\omega - \omega _{\mathrm{o}})^2 + (\varGamma /2)^2}}\) ), and the results are summarized in Fig. 3b–e . The frequencies of the M 1 and M 2 magnons increase slightly, by about 0.8 cm –1 (1.1%) and 3 cm –1 (2.4%), respectively, as the layer number decreases from 13 L to 1 L, possibly because the reduced electronic screening in thinner samples enhances the exchange coupling. In sharp contrast, their lifetimes drop significantly, from about 50 ps (100 ps) in 13 L to 15 ps in 1 L for M 1 (M 2 ), which is consistent with the increased thermal fluctuations in 2D. Despite this decrease, even in the monolayer, the lifetimes are still more than one order of magnitude larger than the corresponding magnon temporal periods, about 30 times for M 1 and 50 times for M 2 . This ratio of magnon lifetime to the temporal period in 2D CrI 3 is significantly higher than that of the Heisenberg ferromagnets [19] , [20] and at least comparable to, if not greater than, that of the antiferromagnets [20] , [21] , [22] , making coherent control of both THz spin waves in the time domain feasible down to the monolayer limit of CrI 3 . Remarkably, I. I. of both magnons, which is known to be proportional to the magnon density, remain nearly constant and independent of the layer number, while that of the phonons scale linearly with the thickness (Fig. 3c, e ). This observation on the M 1 and M 2 magnons is consistent with surface magnons whose density is thickness-independent. 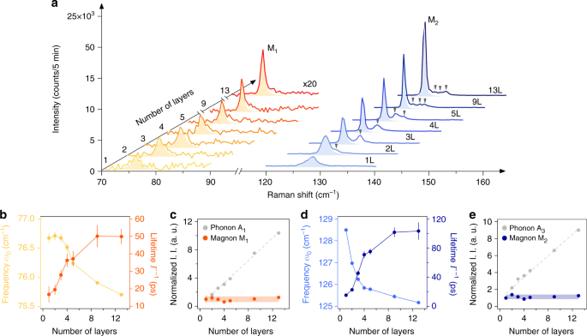Fig. 3 Layer number dependence of the zero-momentum magnon characteristics.aRaman spectra of the M1(intensity multiplied by 20) and M2magnons for 1–5 L, 9 L, and 13 L samples. Light yellow and blue shaded areas are the Lorentzian fits for the M1and M2magnon modes, respectively. The gray triangles highlight the satellite magnon peaks.bFrequency (ω0, left axis) and lifetime (Γ–1, right axis) of the M1magnon as a function of layer number.cI. I. of the M1magnon as a function of layer number with I. I. of the A1phonon shown in gray for comparison.d,ePlots for M2that are similar tob,c, with I. I. of the A3phonon plotted in gray inefor comparison. Error bars inb–erepresent the two SEs of fitting parameters in the Lorentzian fits to individual Raman spectra at different thicknesses Considering that surface magnons have been theoretically predicted in 2D honeycomb ferromagnets [26] , although mainly at different wave vectors K points, it might not be unreasonable to speculate the surface origin of the two THz magnon modes that we have detected here. Phase diagram of 2D CrI 3 By carrying out temperature-dependent Raman measurements and analysis similar to Fig. 2b, c for different thickness samples, we tracked the layer dependence of the 2D ferromagnetism onset temperature. 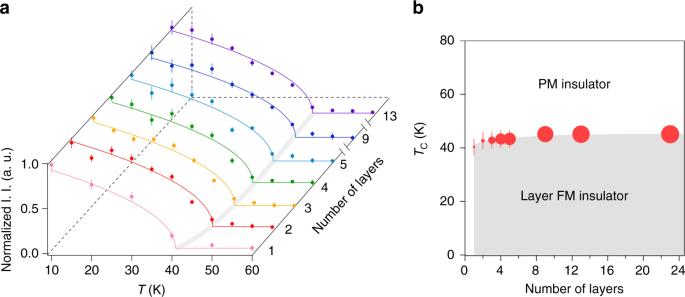Fig. 4 Temperature versus layer number phase diagram of the 2D layer ferromagnetic CrI3.aTemperature dependence of I. I. of the M2magnon normalized to the value at 10 K as a function of layer number. The colored solid curves are fits to\(I_0 + I\sqrt {T_{\mathrm{C}} - T}\). The gray curve is the guide to the eye of the evolution ofTC. Error bars correspond to the two SEs of normalized I. I. in the Lorentzian fits at individual temperatures for different thicknesses of 2D CrI3.bTemperature versus layer number phase diagram (PM for paramagnetism and FM for ferromagnetism). The size of the data points represents the M2magnon lifetime. Error bars correspond to the two SEs ofTCin the fits ina Figure 4a displays the temperature-dependent traces of the normalized I. I. of the M 2 magnon plotted as a function of layer number, with the onset temperature ( T C ) for each trace determined by fitting with an order-parameter-like function for a ferromagnet \({\mathrm{I}}.{\mathrm{I}}. \propto \sqrt {T_{\mathrm{C}} - T}\) (see the similar plot of M 1 in Supplementary Note 6 ). As the layer number decreases from 13 L to 1 L, the extracted T C has an observable decline from 45 K to 40 K. This approximately 12% suppression in T C is in sharp contrast to the slight enhancement of the magnon frequencies, i.e., 1.1% increase of Δ L for M 1 and 2.4% of Δ U for M 2 , which then suggests that the drop in T C is due to stronger thermal fluctuations in thinner samples [35] . Nevertheless, the finite T C for all samples with various thicknesses establishes a phase boundary for the intrinsic transition to the intralayer ferromagnetism in 2D CrI 3 (see Fig. 4b ). Fig. 4 Temperature versus layer number phase diagram of the 2D layer ferromagnetic CrI 3 . a Temperature dependence of I. I. of the M 2 magnon normalized to the value at 10 K as a function of layer number. The colored solid curves are fits to \(I_0 + I\sqrt {T_{\mathrm{C}} - T}\) . The gray curve is the guide to the eye of the evolution of T C . Error bars correspond to the two SEs of normalized I. I. in the Lorentzian fits at individual temperatures for different thicknesses of 2D CrI 3 . b Temperature versus layer number phase diagram (PM for paramagnetism and FM for ferromagnetism). The size of the data points represents the M 2 magnon lifetime. Error bars correspond to the two SEs of T C in the fits in a Full size image We have identified two branches of THz spin waves with their lifetime on the order of 10–100 ps in a 2D Ising ferromagnet, CrI 3 , whose magnetic onset temperature T C remains close to that of their bulk crystal. The robust THz magnons in 2D CrI 3 are in stark contrast to spin waves in conventional metallic ferromagnetic thin films that occur at relatively low, GHz frequencies [16] and also show significant substrate-dependence [36] , [37] , [38] . Similar to many antiferromagnets, 2D CrI 3 is a semiconductor that possesses high-frequency, long-lived spin waves and is free of stray magnetic fields within 2D domains [39] , [40] . Different from bulk antiferromagnets, 2D CrI 3 couples efficiently with external magnetic fields [2] , [3] , [4] , [8] , [11] , [12] and can be tailored in various device geometries with definitive thicknesses [6] , [10] . We envision that these unique characteristics of spin waves in 2D CrI 3 will provide unprecedented opportunities for applications in ultrafast and ultracompact spintronic devices. Magnon dispersion calculations The Ising Hamiltonian with anisotropic exchange coupling is transformed by applying the Holstein–Primakoff transformation. The single-site spin operators, \(S_\phi ^ +\) and \(S_\phi ^ -\) , are related to the momentum space magnon creation and annihilation operators, \(\alpha _{\mathbf{k}}^\dagger\) and α k , as \(S_\phi ^ + = S_\phi ^{\mathrm{X}} + {\mathrm{i}}S_\phi ^{\mathrm{Y}} = \sqrt {2S/N} \mathop {\sum }\limits_{\mathbf{k}} \alpha _{\mathbf{k}}e^{{\mathrm{i}}{\mathbf{k}} \cdot {\mathbf{r}}_\phi }\) , \(S_\phi ^ - = S_\phi ^{\mathrm{X}} - {\mathrm{i}}S_\phi ^{\mathrm{Y}} = \sqrt {2S/N} \mathop {\sum }\limits_{\mathbf{k}} \alpha _{\mathbf{k}}^\dagger e^{ - {\mathrm{i}}{\mathbf{k}} \cdot {\mathbf{r}}_\phi }\) , and \(S_\phi ^{\mathrm{Z}} = S - 1/N\mathop {\sum}\limits_{{\mathbf{k}},{\mathbf{k}}^\prime } {\alpha _{\mathbf{k}}^\dagger \alpha _{{\mathbf{k}}^\prime }e^{{\mathrm{i}}({\mathbf{k}}^\prime - {\mathbf{k}}) \cdot {\mathbf{r}}_\phi }}\) where ϕ = a or b, corresponding to the two Cr 3+ sublattices ( n = 2 and S = 3/2). The bosonic Hamiltonian is then diagonalized using wavefunction \(\psi _{\mathbf{k}} = \left( {\begin{array}{*{20}{c}} {a_{\mathbf{k}}} \\ {b_{\mathbf{k}}} \end{array}} \right)\) to extract the magnon dispersion relations and the eigenvectors. Growth of CrI 3 single crystals The single crystals of CrI 3 were grown by the chemical vapor transport method. Chromium powder (99.99% purity) and iodine flakes (99.999%) in a 1:3 molar ratio were put into a silicon tube with a length of 200 mm and an inner diameter of 14 mm. The tube was pumped down to 0.01 Pa and sealed under vacuum, and then placed in a two-zone horizontal tube furnace. The two growth zones were raised up slowly to 903 K and 823 K for 2 days, and were then held there for another 7 days. Shiny, black, plate-like crystals with lateral dimensions of up to several millimeters can be obtained from the growth. In order to avoid degradation, the CrI 3 crystals were stored in a glovebox filled with nitrogen. Fabrication of few-layer samples CrI 3 samples were exfoliated in a nitrogen-filled glovebox and the thickness of the flakes was first estimated by the optical contrast. Using a polymer-stamping technique inside the glove box, CrI 3 flakes were sandwiched between two few-layer hBN flakes to avoid surface reaction with oxygen and moisture in the ambient environment. The encapsulated CrI 3 samples were then moved out of the glove box for Raman spectroscopy measurements. After Raman spectroscopy measurements, the thicknesses of the encapsulated CrI 3 flakes were determined by the atomic force microscopy (AFM) measurements. Raman spectroscopy Raman spectroscopy measurements were carried out using both a 633-nm and a 532-nm excitation laser with a beam spot size of ~3 μm. The laser power was kept at 80 μW, corresponding to a similar fluence used in literature (10 μW over an ~1-μm-diameter area), to minimize the local heating effect. Backscattering geometry was used. The scattered light was dispersed by a Horiba Labram HR Raman spectrometer and detected by a thermoelectric cooled CCD camera. Selection rule channels XX and XY denote the parallel and cross-polarizations of incident and scattered light at ϕ = 0 o ; X’X’ and X’Y’ represent the parallel and cross-channels at ϕ = 45 o . A closed-cycle helium cryostat was interfaced with the micro-Raman system for the temperature-dependent measurements. All thermal cycles were performed at a base pressure lower than 7 × 10 –7 Torr.